Host factors dictate control of viral replication in two HIV-1 controller/chronic progressor transmission pairs Viremic controllers and elite controllers/suppressors maintain control over HIV-1 replication. Some studies have suggested that control is a result of infection with a defective viral strain, while others suggested host immune factors have a key role. Here we document two HIV-1 transmission pairs: one consisting of a patient with progressive disease and an individual who became an elite suppressor, and the second consisting of a patient with progressive disease and a viremic controller. In contrast to another elite suppressor transmission pair, virus isolated from all patients was fully competent. These data suggest that some viremic controllers and elite suppressors are infected with HIV-1 isolates that replicate vigorously in vitro and are able to cause progressive disease in vivo . These data suggest that host factors have a dominant role in the control of HIV-1 infection, thus it may be possible to control fully pathogenic HIV-1 isolates with therapeutic vaccination. Human immunodeficiency virus-1 (HIV-1) infection is usually characterized by intense viral replication and progressive CD4 + T-cell depletion. However, in defined subsets of infected individuals, the disease course is more benign. Long-term non-progressors are HIV-1-infected individuals who, in the absence of therapy, maintain stable CD4 + T-cell counts greater than 500 cells μl −1 for longer than 7 years. This clinical definition is independent of the level of viremia, which can vary greatly in this subset [1] . Another subset, viremic controllers (VCs), maintain low levels of viremia (<2,000 copies of HIV-1 RNA per ml, detectable by commercially available viral load testing) in the absence of therapy. A third subset, elite suppressors (ES), suppresses viremia to below the clinical limit of detection (50 copies ml −1 ). ES represent <1% of the HIV-1-infected population [1] . Defective or attenuated HIV-1 isolates were initially thought to be responsible for the long-term non-progressor phenotype. Deletions in viral genes such as nef have been shown to facilitate control of HIV-1 infection [2] , [3] , [4] , [5] , [6] , [7] , [8] , [9] , [10] , and rare, stable polymorphisms in HIV-1 isolates from some ES have been documented [11] . It has been hypothesized that these defective isolates may explain the clinical status of these patients. However, it has become increasingly clear that viral factors alone cannot explain the variable nature of HIV-1 infection. Several studies have shown that replication-competent HIV-1 can be isolated from ES [12] , [13] , [14] . Full genome sequence analysis of replication-competent viral isolates from ES revealed no large deletions [12] , and ongoing viral replication and evolution in ES have been documented in recent studies [15] , [16] , [17] . Taken together, these data suggest that, in some cases, infection with attenuated virus cannot explain elite suppression. There is an increasing appreciation for the role played by the host immune response in this phenotype. The HLA-B*57 allele group is overrepresented in ES [18] , [19] , [20] , [21] , [22] , [23] , [24] , and the HIV-1-specific CD8 + T-cell response in these patients is generally superior to that seen in patients with progressive disease [20] , [25] , [26] , [27] . Data supporting a model of host control of viral replication comes from a previous study by our group examining an HIV-1 transmission pair. Virus was transmitted from an HLA-B*57-positive patient who developed AIDS to a recipient who was positive for both HLA-B*57 and HLA-B*27 group alleles and who subsequently became an ES. The viruses infecting both individuals were shown to be closely related by phylogenetic analysis, but the virus isolated from the ES displayed a partial replication defect, and mutations in gag were shown to contribute to this viral attenuation. It was hypothesized that selective pressure from HIV-specific cytotoxic T lymphyocytes (CTLs) caused evolution of the transmitted virus and maintained key escape mutations in HLA-B*27-and HLA-B*57- gag epitopes that resulted in viral attenuation [28] . However, it is possible that selective pressure from the chronic progressors' CD8 + T cells resulted in mutations in HLA-B*57 epitopes early in his disease course. Some of these mutations, such as Gag T242N, have a significant fitness cost [29] , [30] , thus the virus may have been attenuated before transmission, which could have contributed to the elite control of viral replication. We now present two additional HIV-1 transmission pairs each consisting of a patient with progressive disease and a patient who controlled viral replication. These cases differ from the previously reported case because the viruses isolated from all patients were shown to replicate equally well in vitro , suggesting that host factors can control replication of fully pathogenic HIV. Patient characteristics The first transmission pair consists of a 40-year-old male, a chronic progressor (CP1), and a 37-year-old female, a viremic controller (VC1). Infection was first documented in CP1 in 1996, and antiretroviral therapy (ART) was initiated in 1998. The patient had a long history of poor adherence to multiple regimens, and his viral load fluctuated dramatically, as shown in Fig. 1a . CD4 + T-cell counts progressively declined to the current level of 200 cells μl −1 . His partner, VC1, was also diagnosed with HIV-1 infection in 1996. She was originally started on ART for unknown reasons in 1998. Her baseline CD4 + T-cell count was 741 cells μl −1 , and her baseline viral load was 1,184 copies ml −1 . She was taken off treatment in 2000 due to poor adherence ( Fig. 1b ). Since that time, plasma HIV-1 RNA has ranged from <50 to 400 copies ml −1 , and she has maintained an average CD4 + T-cell count of 921 cells μl −1 . 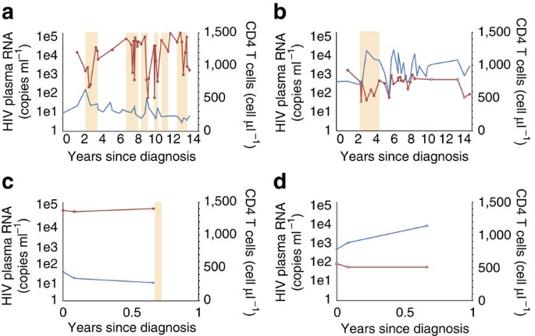Figure 1: Comparison of natural history of infection between transmission pairs. CD4+T-cell counts (blue) and viral load (red) are observed over time for (a) CP1, (b) VC1, (c) CP2 and (d) ES38. Open squares denote viral loads below the limit of detection of the assay. Periods of antiretroviral therapy are indicated by shaded regions for CP1, CP2 and VC1. Figure 1: Comparison of natural history of infection between transmission pairs. CD4 + T-cell counts (blue) and viral load (red) are observed over time for ( a ) CP1, ( b ) VC1, ( c ) CP2 and ( d ) ES38. Open squares denote viral loads below the limit of detection of the assay. Periods of antiretroviral therapy are indicated by shaded regions for CP1, CP2 and VC1. Full size image The second pair consists of a 35–year-old male, a chronic progressor (CP2), and a 21–year- old female who became an ES (ES38). CP2 was found to be infected with HIV-1 in June 2010, and has since maintained plasma HIV-1 RNA levels of approximately 30,000 copies ml −1 . His CD4 + T-cell count reached a nadir of 273 cells μl −1 before initiation of ART ( Fig. 1c ). ES38, who tested negative for HIV-1 in 2008, was also diagnosed with HIV-1 infection in June 2010, but has maintained a plasma HIV-1 RNA level of less than 50 copies ml −1 and an average CD4 + T-cell count of 935 cells μl −1 ( Fig. 1d ). Sequence analysis confirms transmission To confirm transmission of virus between the relevant patients, virus was cultured from each patient's CD4 + T cells with a sensitive coculture assay, as previously described [31] . Full-length sequence analysis was performed, and the resulting genomes were compared with each other and to the consensus B-clade sequence. No large deletions, premature stop codons, frame shifts or other gross defects were seen in the isolates cultured from any of the patients. The number of synonymous nucleotide changes, as well as a number of amino-acid differences, between transmission partners, are shown in Table 1 . Phylogenetic analysis was performed, and full-length env sequences from both transmission pairs were compared with other HIV-1 env sequences obtained from the Los Alamos database ( Fig. 2a ). For both the CP1/VC1 and CP2/ES38 pair, sequences within a pair were more similar to each other than to other B-clade isolates, reflecting a common ancestor consistent with viral transmission within the pairs. Representative sequence alignments ( Fig. 2b ) demonstrate that the sequences within the transmission pairs are closely related. There are rare sequence polymorphisms unique to each transmission pair. Comparative alignments of sequences from CP1 and VC1 revealed unique polymorphisms in tat at nucleotide positions 100 and 101, where aspartic acid (D) is followed by a histadine (H). The combination of these two amino acids at these positions occurs in only 5.3% of B-clade isolates in the Los Alamos HIV sequence database ( Fig. 2b ). This strongly suggests that the two patients are indeed a transmission pair. Similarly, unique polymorphisms were seen in rev and vpu . Unique polymorphisms in tat also confirmed transmission between CP2 and ES38: isolates from both patients had a combination of a phenylalanine (F) followed by a histadine (H) at positions 100 and 101, which is present in <1% of B-clade isolates in the Los Alamos database ( Fig. 2b ). Table 1 Differences in viral isolates in each transmission pair. 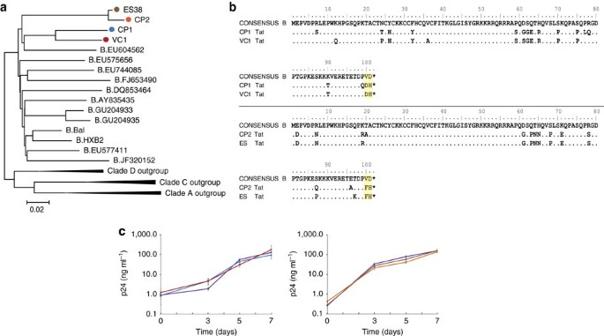Figure 2: Analysis of viral sequences confirms transmission between patients. (a) Phylogenetic tree ofenvsequences from the CP1/VC1 and CP2/ES38 transmission pairs. Phylogenies were estimated by using a 'classical' approach, functioning under maximum-likelihood optimality criterion. Representative B-clade isolates are shown, and A, C and D outgroups are denoted. (b) Tat amino-acid sequences for CP1 and VC1 (top) and Tat amino-acid sequences for CP2 and ES38 (bottom) are compared with consensus B-clade sequence. Rare polymorphisms in Tat, shared within each transmission pair, are highlighted. (c) Fitness of viral isolates from transmission pairs. CD4+T cells from healthy donors were infected, and production of viral p24 was measured over time. Error bars represent standard errors of the means from three independent experiments. On the left, growth kinetics of replication-competent isolates from CP1 (blue) and VC1 (red) are compared with BaL (purple), and on the right growth kinetics of replication-competent isolates from CP2 (orange) and ES38 (brown) are compared with BaL (purple). Full size table Figure 2: Analysis of viral sequences confirms transmission between patients. ( a ) Phylogenetic tree of env sequences from the CP1/VC1 and CP2/ES38 transmission pairs. Phylogenies were estimated by using a 'classical' approach, functioning under maximum-likelihood optimality criterion. Representative B-clade isolates are shown, and A, C and D outgroups are denoted. ( b ) Tat amino-acid sequences for CP1 and VC1 (top) and Tat amino-acid sequences for CP2 and ES38 (bottom) are compared with consensus B-clade sequence. Rare polymorphisms in Tat, shared within each transmission pair, are highlighted. ( c ) Fitness of viral isolates from transmission pairs. CD4 + T cells from healthy donors were infected, and production of viral p24 was measured over time. Error bars represent standard errors of the means from three independent experiments. On the left, growth kinetics of replication-competent isolates from CP1 (blue) and VC1 (red) are compared with BaL (purple), and on the right growth kinetics of replication-competent isolates from CP2 (orange) and ES38 (brown) are compared with BaL (purple). Full size image No significant differences in viral fitness between isolates Previous studies have suggested that attenuation in infecting viruses could explain the clinical outcome of infection [2] , [3] , [4] , [5] , [6] , [7] , [8] , [9] , [10] , [11] . In addition, in a previously reported transmission pair, there was clear viral attenuation in the isolate cultured from the ES, which could have contributed to elite suppression [28] . To determine whether differences in viral fitness could explain the status of both transmission pairs, we isolated replication-competent virus from the latent reservoir of each patient. Multiple isolates were obtained from each patient, and viral replication was compared using healthy donor CD4 + T cells. For the first transmission pair, viral isolates from VC1 were as fit as isolates from CP1 ( Fig. 2c ). The second transmission pair showed similar results, with no differences in viral fitness seen in isolates cultured from CP2 and ES38 ( Fig. 2c ). All viral isolates replicated as efficiently as the HIV-1 BAL reference strain. The role of host factors in the control of viral replication As no differences were seen in the replication of viruses from each member of the two transmission pair, and as all viruses were as fit as the reference strain HIV-1 BaL , we sought to determine whether cellular factors could be having a predominant role in determining the clinical phenotype. Subjects who are heterozygous for the delta 32 mutation in CCR5 have slower progression of HIV-1 disease [32] . The CCR5 gene was analysed by PCR, and all patients were determined to have two wild-type CCR5 alleles. Human leukocyte antigen (HLA)-typing was also performed on each patient. It is interesting to note that ES38 is HLA-B*57:03 positive. This is a protective allele group that is overrepresented in ES [18] , [19] , [20] , [21] , [22] , [23] , [24] . No known protective HLA alleles were present in VC1, CP1 or CP2 ( Table 2 ). A single-nucleotide polymorphism (SNP) associated with the HLA-C promoter (rs9264942) has also been implicated in the control of viral replication in a genome-wide association study [33] . Of the four patients, none were homozygous for the protective allele ( Table 2 ). Table 2 Cellular factors of viral control. Full size table Natural killer (NK) cells have been implicated in delaying the progression of HIV-1 disease. The interaction between the NK cell receptor KIR3DS1 and HLA-Bw4-80Ile motif has been shown to be protective [34] . We sought to determine whether our patients possessed this protective combination. None of our patients were positive for the KIR3DS1 -activating allele ( Table 2 ), and only ES38 was positive for an HLA-B Bw4-80Ile motif. CD8 + T-cell response in ES To determine how pressure from HIV-1-specific CTL responses might have led to differences in viral evolution in the patients, we performed interferon (IFN)-γ enzyme-linked immunosorbent spot (ELISPOT) assays to determine which epitopes were targeted in Gag and Nef. The epitope DQ15 (Gag 219–233) was targeted by both CP1 and VC1, but mutations in this region were observed only in isolates from CP1 ( Fig. 3 ). Similarly, a mutation was present in NP15 (Gag 331–346), an epitope targeted by VC1, indicating potential virologic escape in this subject. 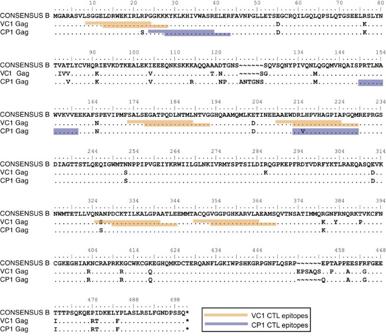Figure 3: Gag sequences from VC1 and CP1. Patient-specific CTL epitopes were identified by IFN-γ ELISPOT, and are highlighted for each patient. Numbering indicates amino-acid position in Consensus B-Clade Gag. Figure 3: Gag sequences from VC1 and CP1. Patient-specific CTL epitopes were identified by IFN-γ ELISPOT, and are highlighted for each patient. Numbering indicates amino-acid position in Consensus B-Clade Gag. Full size image CP2 and ES38 each targeted several epitopes in Gag ( Fig. 4 ). Interestingly, ES38 made responses to peptides that contained previously characterized HLA-B*57-restricted epitopes, and both ES38 and CP2 had mutations in HLA-B*57-restricted Gag and Nef epitopes, including L90V and H121N in Nef and I147L, G248A, I247V and E312D in Gag. In addition, an S173T mutation that has been seen in HLA-B*57 individuals [35] was present adjacent to the immunodominant HLA-B*57-restricted KF11 epitope (gag 162–172) in both patients. The presence of these mutations in both patients, including CP2 who is not positive for HLA-B*57 ( Table 2 ), would suggest that either CP2 was originally infected with virus from an HLA-B*57-positive patient, or that ES38 transmitted virus to CP2 after these mutations developed. Phylogenetic analysis of clonal nef sequences ( Fig. 5a ) amplified from resting CD4 + T cells from both patients was performed, but the results could not definitively distinguish between the two hypotheses. 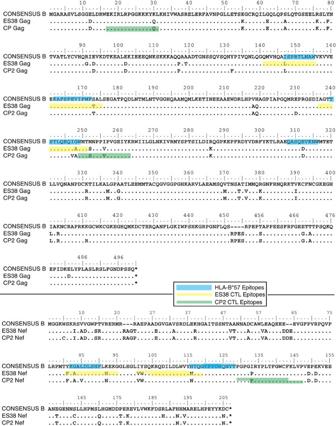Figure 4: Gag and Nef Sequences from CP2 and ES38. Patient-specific CTL epitopes were identified by IFN-γ ELISPOT, and are highlighted for each patient. HLA-B*57-restricted epitopes are indicated. Numbering indicates amino acid position in consensus B-clade Gag or Nef. Figure 4: Gag and Nef Sequences from CP2 and ES38. Patient-specific CTL epitopes were identified by IFN-γ ELISPOT, and are highlighted for each patient. HLA-B*57-restricted epitopes are indicated. Numbering indicates amino acid position in consensus B-clade Gag or Nef. 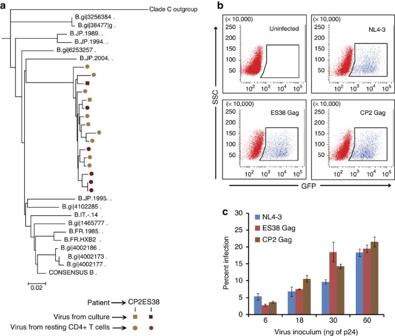Figure 5: Phylogenetic analysis andgagfitness in virus from ES38 and CP2. (a) Phylogentic tree of clonalnefsequences isolated from resting CD4+T cells (circles) and replication-competent virus isolates for reference. Phylogenies were estimated by using a 'classical' approach, functioning under maximum-likelihood optimality criterion. Other representative B-clade isolates, consensus B-cladenefand the clade C outgroup are denoted. Fitness of patient-specific viralgag. (b) Representative fluorescence-activated cell sorting plots showing GFP expression indicates infection with single cycle, pseudotyped virus. (c) Percent infection with various volumes of pseudotyped virus containinggagfrom ES38 (red), CP2 (brown) and wild-type NL4-3 (blue) was determined and repeated for three donors, producing similar results. Approximate levels of p24 in each infectious volume are shown, estimated and normalized based on NL4-3. Infection of healthy donor CD4+T cells was normalized by transfection efficiency. Error bars represent standard error of the means from three independent experiments. Full size image Figure 5: Phylogenetic analysis and gag fitness in virus from ES38 and CP2. ( a ) Phylogentic tree of clonal nef sequences isolated from resting CD4 + T cells (circles) and replication-competent virus isolates for reference. Phylogenies were estimated by using a 'classical' approach, functioning under maximum-likelihood optimality criterion. Other representative B-clade isolates, consensus B-clade nef and the clade C outgroup are denoted. Fitness of patient-specific viral gag . ( b ) Representative fluorescence-activated cell sorting plots showing GFP expression indicates infection with single cycle, pseudotyped virus. ( c ) Percent infection with various volumes of pseudotyped virus containing gag from ES38 (red), CP2 (brown) and wild-type NL4-3 (blue) was determined and repeated for three donors, producing similar results. Approximate levels of p24 in each infectious volume are shown, estimated and normalized based on NL4-3. Infection of healthy donor CD4 + T cells was normalized by transfection efficiency. Error bars represent standard error of the means from three independent experiments. Full size image It has been shown that some escape mutations in HLA-B*57-restricted epitopes in Gag have a negative effect on viral fitness [15] , [30] and may contribute to elite control. ES38 did not possess the T242N mutation, which is known to revert when transmitted to HLA-B*57-negative individuals [36] , [37] , [38] . Nonetheless, to determine whether other mutations in this gene had significant effects on fitness, we cloned the gag genes from CP2 and ES38 and compared infection of healthy donor CD4 + cells with these isolates to infection with NL4-3. There was no significant difference in the infectivity of virus expressing patient-derived Gag ( Fig. 5b,c ). Thus, the difference in the level of viral control in these patients cannot be attributed to differences in viral fitness. In addition, the infection levels of both viruses was similar to that of the reference strain, further suggesting that ES38 was exerting control over a virus that replicates as well in vitro as does virus from a patient with progressive disease. Taken together, these data suggest that viral fitness is not the determining factor that explains differences in the clinical outcome seen in the patients in both of the reported transmission pairs. ES38 was positive for the HLA-B*57 allele, which has been associated with elite control of HIV-1 replication in many studies. However, VC1 does not have any known protective HLA alleles; therefore, we compared multiple aspects of her HIV-1-specific immune response to those seen in CP1. As shown in Fig. 6a , stimulation of peripheral blood mononuclear cells (PBMCs) with overlapping Gag peptides resulted in a substantially higher percentage of IFN-γ-expressing HIV-specific CD4 + T cells that coexpressed interleukin (IL)-2 in VC1 compared with CP1, consistent with previous studies showing the preservation of IL-2 secretion in aviremic individuals [39] , [40] , [41] , [42] . CD8 + T-cell responses have been intensely studied in ES. It has been shown that CTLs from ES are more likely to upregulate cytolytic granules containing perforin and granzyme B [20] , [25] , [27] . These cells are also more likely to coexpress IFN-γ and tumour necrosis factor (TNF)-α [43] , which is a known correlate of cytotoxic activity [44] . IFN-γ-expressing HIV-specific CD8 + T cells from VC1 fit this profile and coexpressed more perforin and TNF-α in response to stimulation with Gag and Nef peptides than did CD8 + T cells from CP1 ( Fig. 6b–d ). To determine whether this phenotype was associated with actual inhibition of viral replication, a suppression assay was performed. Because CP1 was on HAART, CD4 + T cells from both patients were incubated for a week before infection with pseudotyped virus. Freshly isolated CD8 + T cells from CP1 had no effect on CD4+ T-cell infection, whereas CD8+ T cells from VC1 substantially reduced the percentage of infected cells ( Fig. 6e ). In a traditional inhibition assay where there was no preincubation of CD4+ T cells before stimulation and infection, CD8 + T cells of VC1 were seen to be as effective as those from a cohort of HLA-B*57 ES in controlling replication-competent virus in vitro , whereas CD8 + T cells from patients with progressive disease and uninfected individuals had low inhibitory activity ( Fig. 6f ). 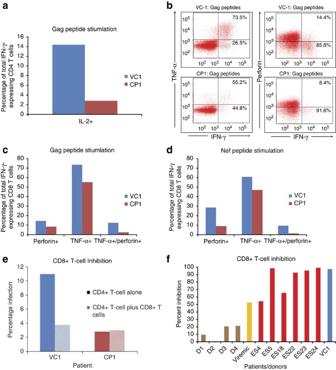Figure 6: Differential HIV-specific CD4+T-cell and CD8+T-cell cytokine response. (a) Stimulation of patient PBMCs cells isolated directlyex vivowith overlapping Gag peptides. The percent of IFN-γ-expressing HIV-specific CD4+T cells that coexpressed IL-2 is shown for VC1 and CP2. A minimum of 250,000 total events were analysed by fluorescence-activated cell sorting (FACS). (b) Representative FACS plots showing the stimulation of PBMCs isolated from VC1 and CP1. The plots are gated on all CD8+T cells, and the percentage of IFN-γ-positive cells that coexpressed TNF-α or perforin are indicated in the top right quadrant. Quantification of the percentage of IFN-γ-expressing CD8+T cells that coexpressed perforin, TNF-α or both perforin and TNF-α after stimulation with patient-specific Gag (c) or Nef (d) peptides are shown for both VC1 and CP1. A minimum of 250,000 total events were analysed by FACS. Comparative CD8+T-cell inhibition of viral replication. (e) CD4+T cells from VC1 and CP1 were infected with GFP-expressing recombinant NL4-3 virus. CD4+T-cells were cultured alone or with autologous CD8+T cells at a 1:1 ratio. Percent infection was measured 5 days after infection by FACS analysis. (f) CD4+T cells from four healthy donors (D1–4), an untreated Viremic patient, six ES and VC1 were infected with GFP-expressing replication-competent NL4-3 virus. CD4+T cells were cultured alone or with autologous CD8+T cells at a 1:1 ratio. Percent inhibition was quantified 5 days after infection. Figure 6: Differential HIV-specific CD4 + T-cell and CD8 + T-cell cytokine response. ( a ) Stimulation of patient PBMCs cells isolated directly ex vivo with overlapping Gag peptides. The percent of IFN-γ-expressing HIV-specific CD4 + T cells that coexpressed IL-2 is shown for VC1 and CP2. A minimum of 250,000 total events were analysed by fluorescence-activated cell sorting (FACS). ( b ) Representative FACS plots showing the stimulation of PBMCs isolated from VC1 and CP1. The plots are gated on all CD8 + T cells, and the percentage of IFN-γ-positive cells that coexpressed TNF-α or perforin are indicated in the top right quadrant. Quantification of the percentage of IFN-γ-expressing CD8 + T cells that coexpressed perforin, TNF-α or both perforin and TNF-α after stimulation with patient-specific Gag ( c ) or Nef ( d ) peptides are shown for both VC1 and CP1. A minimum of 250,000 total events were analysed by FACS. Comparative CD8 + T-cell inhibition of viral replication. ( e ) CD4 + T cells from VC1 and CP1 were infected with GFP-expressing recombinant NL4-3 virus. CD4 + T-cells were cultured alone or with autologous CD8 + T cells at a 1:1 ratio. Percent infection was measured 5 days after infection by FACS analysis. ( f ) CD4 + T cells from four healthy donors (D1–4), an untreated Viremic patient, six ES and VC1 were infected with GFP-expressing replication-competent NL4-3 virus. CD4 + T cells were cultured alone or with autologous CD8 + T cells at a 1:1 ratio. Percent inhibition was quantified 5 days after infection. Full size image Understanding the mechanisms of control of viral replication in VC and ES may lead to effective immunotherapy of HIV-1 infection. Determining the role of viral fitness versus host factors in these patients is critical, because it bears directly on the fundamental mechanism of elite control of HIV-1 replication. Unfortunately, isolating replication-competent virus from ES has proven to be extremely challenging. As a result, many studies have focused on the analysis of proviral and/or plasma sequences from ES. Some studies have not found any deleterious mutations or large deletions [45] , [46] , whereas others have reported significant deletions [2] , [3] , [4] , [5] , [6] , [7] , [8] , [9] , [10] , [11] and/or reductions in the fitness of recombinant viruses expressing viral genes amplified from ES [46] , [47] , [48] , [49] . The results of these studies are limited by the fact that many proviral clones are not replication competent and the viruses in the plasma of ES typically contain attenuating escape mutations not found in virus archived in resting CD4+ T cells [50] . Full genome sequence analysis has been performed for less than ten replication-competent isolates cultured from ES CD4 + T cells [11] , [12] , [28] , [51] , and there has been only one documented case of viral transmission from a CP to an ES described in the literature [28] . The two transmission pairs presented here are unique because they stand in contrast to the previously reported transmission pair: in this study, viruses isolated from both VC1 and ES38 were fully replication competent and as fit as viruses isolated from their partners with progressive HIV-1 disease. In the previous study, the ES was found to have an attenuated viral isolate. While we hypothesized that the diminished fitness in this patient was due to escape mutations that developed in response to strong selective pressure from CTL, it is also possible that viral attenuation preceded transmission and contributed to ES [28] . However, in this report, we have shown for the first time that replication-competent isolates obtained from patients who controlled viral replication had no evidence of attenuation and had the potential to cause progressive disease in vivo . This strongly suggests that in some cases elite suppression is not the result of infection with attenuated viruses. While ES38 is HLA-B*57:03 positive, no other known cellular factors could explain viral control in either of these transmission pairs. The HLA-C-related SNP and the delta 32 CCR5 mutation that confer relative protection against HIV-1 infection were not present in any of our patients, and all patients lacked the combination of KIR3DS1 and protective HLA-B alleles. CD8 + T cells have been extensively studied in control of HIV-1 infection, and strong evidence supports their key role in delaying disease progression [20] , [25] , [26] , [27] . While we were unable to perform detailed HIV-specific CD8 + T-cell analysis in ES38 due to a lack of cells, it is likely that HIV-specific HLA-B*57-restricted CTL had a role in elite control of viral replication. VC1 did not have any known protective HLA allele, but, unlike CP1, she had polyfunctional HIV-specific CD4 + T cells, and her HIV-specific CD8 + T cells expressed substantial levels of perforin and TNF-α on activation and were as effective at inhibiting HIV-1 replication as CD8+ T cells from many HLA-B*57-positive ES. Thus, the differences in CD8 + T-cell function can probably explain the difference in clinical outcomes seen in these patients. These data support the hypothesis that ES are infected with virus that replicates as well as virus that causes progressive disease, and a combination of host immune factors, unique to ES, enables control of viral replication. While infection with an attenuated virus can increase the chance of early and prolonged control of viral replication, this study and others supports a model in which host factors have a dominant role in determining the clinical outcome of infection. These results are consistent with the macaque model of elite control, in which animals with protective major histocompatibility complex alleles are capable of controlling fully replication-competent laboratory strains of SIV (reviewed in ref. 52 ). Intriguingly, in two distinct elite monkey models, depletion of CD8 + T cells with monoclonal antibodies results in the transient loss of control of viral replication [53] , [54] , implying that these cells have a major role in elite suppression. Importantly, these data suggest that ESs have a unique capacity to restrict viral replication, independent of the fitness of the infecting virus. Our sequence analysis suggests that ES31 may have infected CP2 who then went on to develop a rapid decline in his CD4 + T-cell count. Overall, the data presented here provide the strongest evidence to date that in some cases host factors rather than viral fitness determine clinical outcome. Thus, by identifying the contribution of individual host factors, the mechanism of elite suppression could form the basis for a therapeutic vaccine for HIV-1. Patient consent All patients were provided written, informed consent, and the handling of all patient samples was in accordance with the policies dictated by the Johns Hopkins University regulations. Virus isolation and sequence analysis Culture of replication-competent virus and full genome sequence analysis of proviral and plasma virus were performed using a modified, highly sensitive coculture assay [12] . Clonal nef sequences were amplified from resting CD4+ T cells as previously described [16] . Classical, maximum likelihood and Bayesian phylogenetic analysis were performed as described previously [15] . The nested primers used in the study are as follows: LTR1 out (5′-cacacaaggctayttccctga-3′), LTR2 out (5′-TCCYCYTGGCCTTAACCGAAT-3′); LTR3 inner (5′-ACTGTCTAGATGGATGGTGCTWCAAGYTAGT-3′), LTR4 inner (5′-ACTGCTCGAGTCCTTCTAGCCTCCGCTAGTC-3′); 5 gag Outer (5′-GCGAGAGCGTCAGTATTAAGC-3′), 3 gag outer (5′-TCTTTATCTAAGGGAACTGAAAAATATGCATC-3′); 5 gag In (5′-GGGAAAAAATTCGGTTAAGGCC-3′), 3 gag In (5′-CGAGGGGTCGTTGCCAAAGA-3′); 5 outer FL (5′-GCCCCTAGGAAAAAGGGCTGTTGG-3′), 3 outer FL (5′-CCTTGCCCCTGCTTCTGTATTTCTGC-3′); 5 inner FL (5′-TGCAGGGCCCCTAGGAAAAAGGGCTG-3′), 3 inner FL (5′-CATGTACCGGTTCTTTTAGAATCTCCCTGT-3′), 5 integrase outer (5′-ACTCCATCCTGATAAATGGACAG-3′), 3 integrase outer (5′-AATCCTCATCCTGTCTACTTGCC-3′); 5 integrase inner (5′-GAAAATTGAATTGGGCAAGTC-3′), 3 integrase inner (5′-CCACACAATCATCACCTGCC-3′); accessory outer 1 (5′-CGGGTTTATTACAGGGACARCARA-3′), accessory outer 2 (5′-GGCATGTGTGGCCCARAYATTAT-3′); accessory inner 1 (5′-GGTGAAGGGGCAGTAGTAATACAA-3′), accessory inner 2 (5′-CCCATAATARACTGTGACCCACAA-3′); 5 Env outer (5′-ATGGCAGGAAGAAGCGGAGACAG-3′), RT4.2 (5′-GCTCAACTGGTACTAGCTTGAAGCACC-3′); 5 Env inner (5′-GATAGACGCGTAGAAAGAGCAGAAGACAGTGGCAATG-3′), 3 Env inner (5′-CCTTGTGCGGCCGCCTTAAAGGTACCTGAGGTCTGACTGG-3′); 5 Nef outer (5′-GTAGCTGAGGGGACAGATAGGGTTAT-3′), 3 Nef outer (5′-GCACTCAAGGCAAGCTTTATTGAGGC-3′); 5 Nef inner (5′-CGTCTAGAACATACCTAGAAGAATAAGACAGG-3′), 3 Nef inner (5′-CGGAATCCGTCCCCAGCGGAAAGTCCCTTGTA-3′). Viral fitness assay Viral fitness was analysed as described previously [12] . PBMCs from healthy donors were cultured for 2 days in the presence of IL-2 and phytohaemagglutinin. CD4+ T cells were isolated (MACS, CD4+ T cell isolation Kit) and infected by spinoculation [55] (1,200 g for 2 h) with equal quantities (200 ng ml −1 ) of p24 from primary patient isolates, and with HIV-1 BAL as a reference strain. Supernatant samples were taken over the course of 7 days. Viral replication was quantified using p24 ELISA (Perkin Elmer). To study the effect of mutations in HLA-B*57 epitopes on gag fitness, gag from patient viral isolates was amplified by PCR. The resulting amplicon was digested with BSS HII and Sbf I restriction enzymes and ligated into a previously described pNL4-3-ΔEnv GFP NL43dE vector [56] . The pNL4-3-ΔEnv GFP NL43dE vector with patient-specific gag was transformed into Stbl-3 cells (Invitrogen) to amplify, and co-transfected into 293T cells with an X4 Env plasmid to produce single round replication pseudovirus expressing patient-specific gag . After a 3-day transfection, cellular debris was removed by centrifugation and filtration through Steriflip filters (Millipore). Virus was collected by ultracentrifugation at 1,200 g for 2 h at 25 °C. CD4 + T cells from healthy donor PBMCs were isolated by magnetic bead separation (Miltenyi), and were infected by spinoculation with NL4-3 (control), ES31- gag and CP2- gag pseudoviruses. Infection was analysed after 3 days of infection by measuring green fluorescent protein (GFP) expression using a flow cytometer. The results were normalized by transfection efficiency. Genetic polymorphisms HLA-A and HLA-B locus allele identification was performed as previously described [12] . CCR5 from all patients was amplified from genomic DNA using gene-specific primers. The presence or absence of the CCR5 Δ32 mutation was determined by relative size of the resulting PCR fragment. HLA-C SNP genotyping (rs9264942) was performed using the Applied Biosystems 7300 real-time PCR System allelic discrimination assay (Applied Biosystems), following the manufacturer's guidelines. Primers and probes were developed by Custom TaqMan SNP Genotyping assays (ABI). Determination of the KIR3DS1 and HLA-B Bw4-80Ile allele was performed using the Olerup SSP 104.101 KIR Genotyping 12 Lot71E and 104.201 KIR ligand genotyping Lot85E kits, following the manufacturer's guidelines. Immunologic assays Cytokine expression was determined by an intracellular cytokine staining assay as previously described [28] . PBMCs were stimulated overnight with either HIV-1 Gag Nef peptides at a concentration of 5 μg ml −1 . For CD8 + T-cell analysis, patient-specific Gag or Nef peptides determined by IFN-γ ELISPOT were used. For CD4 + T-cell cytokine analysis, overlapping peptides spanning the entire amino-acid sequence of B-clade consensus Gag were used. Conjugated antibodies specific for perforin (Diaclone Research), IL-2 (BD Biosciences), INF-γ (BD Biosciences) and TNF-α (BioLegend) were used to examine cytokine expression by flow cytometry. The Cytolytic T-cell effect for VC1 compared with healthy donors, viremic patients and ES was determined by a CD8 suppression assay. PBMCs were isolated from patients, and CD8 + T cells were positively selected using Miltenyl magnetic beads (MACS, CD8+ T cell Isolation kit). CD8 + T cells were depleted of CD16 + cells (Invitrogen, Dynal Beads) to remove contaminating NK cells. CD4 + T cells were isolated by negative selection using Miltenyi magnetic beads. Purity of depletion was analysed by flow cytometry. CD4 + T cells were infected by spinoculation at 1,200 g for 2 h with replication-competent NL4-3 virus, in which GFP is engineered into nef . Autologous CD8 + T cells were added at a 1:1 ratio to CD4 + T cells, and infection between cultures with and without CD8 + T-cell addition were compared. Fluorescence-activated cell sorting analysis was performed 5 days after infection. To compare cytolytic T-cell effects between VC1 and CP1, PBMCs were isolated and cultured for 3 days in stimulating media. CD4 + T cells were isolated after 3 days, and maintained in stimulating media for another 4 days to diminish the inhibitory effect of the antiretroviral drugs that CP1 was on. The CD4 + T cells were spinoculated at 1,200 g for 2 h with single-cycle pseudotyped NL4-3 virus. This virus was used to minimize the differences in the amount of replication that occurred in the patients' CD4 + T cells. Autologous CD8 + T cells, isolated directly ex vivo , were added at a 1:1 ratio to CD4 + T cells, and infection between cultures with and without CD8 + T-cell addition. Fluorescence-activated cell sorting analysis was performed 5 days after infection. To produce the replication-competent NL4-3, the pNL4-3-ΔNef GFP vector was transformed into Stbl-3 cells (Invitrogen) to amplify, and transfected into 293T cells to produce pseudovirus. After a 3-day transfection, cellular debris was removed by centrifugation and filtration through Steriflip filters (Millipore). Virus was collected by ultracentrifugation at 1,200 g for 2 h at 25 °C. To produce the single-cycle NL4-3, the pNL4-3-ΔEnv GFP NL43dE vector was transformed into Stbl-3 cells (Invitrogen) to amplify, and co-transfected into 293T cells with an X4 Env plasmid to produce single round replication pseudovirus. After a 3-day transfection, cellular debris was removed by centrifugation and filtration through Steriflip filters (Millipore). Virus was collected by ultracentrifugation at 1,200 g for 2 h at 25 °C. Reactive CTL epitopes were defined by IFN-γ ELISPOT. As previously described [28] , whole blood was taken from each patient and PBMCs were isolated by Ficoll gradient centrifugation. PBMCs were aliquoted into each well of 96-well MultiScreen (Millipore) plates with conjugated IFN-γ antibody. Cells were activated with overlapping peptides spanning the entire amino-acid sequence of B-clade consensus gag and nef . Alternatively, cells were activated with peptides representing conserved epitopes in HLA-B*57. PBMCs were cultured overnight, and subsequently analysed. Quantification of spot-forming units was performed independently and in a blinded manner. Nucleotide sequences accession numbers Full genome sequences from each patient have been submitted to the nucleotide core GenBank database and have been assigned accession numbers JN397362 to JN397365 . Accession codes: Sequence data have been deposited in the nucleotide core GenBank database under accession codes JN397362 to JN397365 . How to cite this article: Buckheit, R.W. III et al . Host factors dictate control of viral replication in two HIV-1 controller/chronic progressor transmission pairs. Nat. Commun. 3:716 doi:10.1038/ncomms1697 (2012).